Covalently linked hopanoid-lipid A improves outer-membrane resistance of aBradyrhizobiumsymbiont of legumes Lipopolysaccharides (LPSs) are major components of the outer membrane of Gram-negative bacteria and are essential for their growth and survival. They act as a structural barrier and play an important role in the interaction with eukaryotic hosts. Here we demonstrate that a photosynthetic Bradyrhizobium strain, symbiont of Aeschynomene legumes, synthesizes a unique LPS bearing a hopanoid covalently attached to lipid A. Biophysical analyses of reconstituted liposomes indicate that this hopanoid-lipid A structure reinforces the stability and rigidity of the outer membrane. In addition, the bacterium produces other hopanoid molecules not linked to LPS. A hopanoid-deficient strain, lacking a squalene hopene cyclase, displays increased sensitivity to stressful conditions and reduced ability to survive intracellularly in the host plant. This unusual combination of hopanoid and LPS molecules may represent an adaptation to optimize bacterial survival in both free-living and symbiotic states. Hopanoids, pentacyclic triterpenoids, constitute an important class of membrane lipids widely distributed in diverse bacteria [1] , [2] , [3] . These molecules, used by geobiologists as ‘biomarkers’ to assess patterns of bacterial distribution in both ancient and modern ecosystems [4] , display structural similarity with eukaryotic sterols [5] . Hopanoids are thought to stabilize membranes, control fluidity and permeability and bolster the integrity of bacterial cell envelope [6] . Lipopolysaccharides (LPSs) are components of the outer membrane of Gram-negative bacteria. Their structural and functional properties are diverse, ranging from restricting the permeability of the outer membrane to playing a central role in bacterial invasion and adaptation to the host environment [7] , [8] . The general structure of LPS consists of a hydrophilic portion composed of a distal polysaccharide, which in most cases represents the O-antigen, and a proximal oligosaccharide, termed the core, which, in turn, is linked to a glycolipid moiety named lipid A. Noteworthy, in both mammal and plant cells, lipid A is responsible for the interaction with host receptors [7] . Rhizobia are Gram-negative soil bacteria that can establish a symbiotic relationship with legumes, where the bacteria provide the plant with a source of nitrogen [9] , [10] . Their ability to fix nitrogen from natural sources holds promise as a viable alternative to the use of industrial N-fertilizer in agriculture [11] , [12] . In rhizobia, LPSs play a role throughout the symbiotic process and their structures are altered in response to plant signals [8] , [13] . The remarkable structural diversity in the O-antigen region observed among rhizobial species is believed to be a strategy to modulate or suppress plant defence responses, thus facilitating the establishment of symbiosis [14] . Furthermore, the lipid A of rhizobial LPS, characterized by a peculiar lipid and sugar composition and by the presence of very long-chain fatty acids (VLCFA), is important in their adaptation to the intracellular life [14] , [15] , [16] . Photosynthetic bradyrhizobia elicit nitrogen-fixing nodules on roots and stems of some tropical legumes belonging to the Aeschynomene genus. Unlike other rhizobia, they lack the canonical nodABC genes required for the synthesis of Nod factors (NFs), the signal molecules that initiate symbiosis and which had been thought to be universal to all rhizobium–legume interactions [17] . This finding suggests alternative symbiotic strategies and different molecular patterns involved in NF-independent symbiosis, in which the LPS might play an important role. Previously, we showed that the Nod-independent Bradyrhizobium BTAi1 strain suppresses basal defence in plants through an LPS composed of a unique monosaccharide [18] . In the present study, we demonstrate that BTAi1 also builds a unique LPS lipid A that is covalently substituted by a hopanoid structure. In addition, BTAi1 produces other hopanoids that are not linked to LPS. By constructing a hopanoid-deficient mutant, we show that hopanoids are essential for both free-living and symbiotic life of the bacteria. Structure of the lipid A from Bradyrhizobium BTAi1 The primary structure and the supramolecular arrangement of the lipid A isolated from BTAi1 were obtained using mass spectrometry (MS), nuclear magnetic resonance (NMR) spectroscopy, electron spin resonance (ESR) spectroscopy and dynamic light scattering (DLS). These different analytical methods revealed the presence of a novel hopanoid molecule as an LPS constituent. Representative depictions of this unique lipid A structure (compound 1 ) are illustrated in Figs 1 and 2 ; further details on the in-depth characterization are presented in Supplementary Notes 1–4 and Supplementary Tables 1–3 . 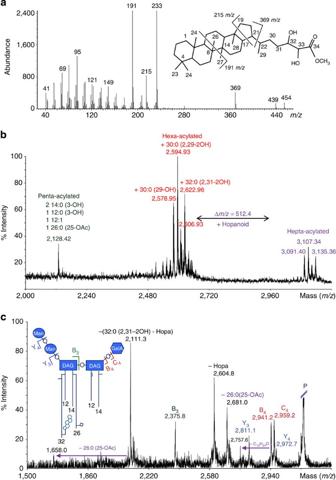Figure 1: MS analysis ofBradyrhizobiumBTAi1 lipid A. (a) Mass spectrum of carboxy-methylated hopanoid derivative as obtained by GC-MS analysis of the lipid A; the hopanoid numbering and fragmentation pattern are reported in the inset. (b) Reflectron MALDI TOF mass spectrum in positive ion more of the lipid A fromBradyrhizobiumBTAi1; ion peaks are present as Na+adducts. (c) MALDI TOF/TOF MS2analysis of the hepta-acylated lipid A species atm/z3135.36 (P: parent ion). The lipid A is sketched, letters refer to the ions generated in the MS/MS spectrum. The square indicates the acetyl group, the hopanoid is schematically indicated with the pentacyclic triterpenoid moiety (DAG, 2,3-diamino-2,3-dideoxy-D-glucopyranose; GalA, galacturonic acid; Man, mannose; Hopa, hopanoid). Figure 1: MS analysis of Bradyrhizobium BTAi1 lipid A. ( a ) Mass spectrum of carboxy-methylated hopanoid derivative as obtained by GC-MS analysis of the lipid A; the hopanoid numbering and fragmentation pattern are reported in the inset. ( b ) Reflectron MALDI TOF mass spectrum in positive ion more of the lipid A from Bradyrhizobium BTAi1; ion peaks are present as Na + adducts. ( c ) MALDI TOF/TOF MS [2] analysis of the hepta-acylated lipid A species at m/z 3135.36 (P: parent ion). The lipid A is sketched, letters refer to the ions generated in the MS/MS spectrum. The square indicates the acetyl group, the hopanoid is schematically indicated with the pentacyclic triterpenoid moiety (DAG, 2,3-diamino-2,3-dideoxy- D -glucopyranose; GalA, galacturonic acid; Man, mannose; Hopa, hopanoid). 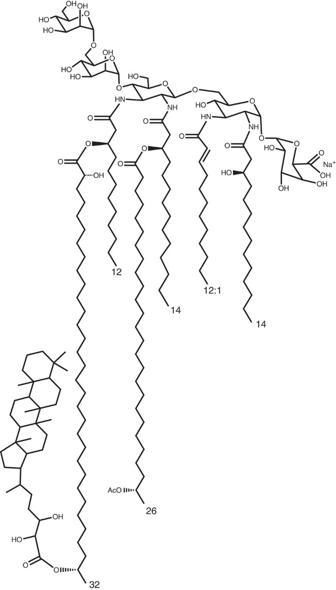Figure 2:BradyrhizobiumBTAi1 lipid A structure. BradyrhizobiumBTAi1 lipid A structure of the hepta-acylated ion species atm/z3,135.36 (compound1). Full size image Figure 2: Bradyrhizobium BTAi1 lipid A structure. Bradyrhizobium BTAi1 lipid A structure of the hepta-acylated ion species at m/z 3,135.36 (compound 1 ). Full size image Briefly, the positive ion matrix-assisted laser desorption ionization (MALDI) spectrum of lipid A ( Fig. 1b ) exhibited a heterogeneous mixture of ion peaks, present as Na + adducts, belonging to three families of molecules differing in their acylation pattern, namely, in the lipid chain nature and content; for each family, the mass differences between neighbouring ions were due to the different lengths and/or substitution patterns of the ester-linked acyl chains ( Supplementary Note 3 , Supplementary Figs 1–3 ). The lowest molecular mass peak at m/z 2,128.42 was identified as a penta-acylated form possessing two 14:0(3-OH), one 12:0(3-OH) one 12:1 and one acetylated VLCFA, 26:0(25-OAc); no additional peaks were observed in this mass range. The mass peak at m/z 2,622.96 carried an additional secondary VLCFA recognized as 32:0(2,31-2OH). The third lipid A ion cluster showed an analogous acylation pattern shifted at higher molecular mass by Δ m/z 512.4. The mass difference (fit with a molecular formula C 34 H 56 O 3 ) matched the hopanoid residue identified using GC-MS and NMR analyses. MS/MS analysis of the ion species at m/z 3,135.36 ( Figs 1c and 2 , Supplementary Note 3 ) indicated that the hopanoid moiety was a tertiary substituent, located at the ω-1 position of the long-chain fatty acid as deduced using NMR. This latter approach (see Supplementary Note 4 , Supplementary Table 2 and Supplementary Figs 4–7 ) allowed us to establish the full structure of lipid A from BTAi1 ( Fig. 2 ). It consisted of an invariable pentasaccharide sugar backbone formed by a skeleton of β-(1→6)-linked 2,3-diamino-2,3-dideoxy- D -glucopyranose (DAG) carrying an α-Gal p A on the vicinal DAG and an α-(1→6) Man p disaccharide on the distal DAG unit, substituted by a heterogeneous blend, in terms of number and nature, of lipid chains asymmetrically distributed on the sugar skeleton. The two secondary VLCFAs were substituted by a hopandiolic acid and by an acetyl group. Interestingly, of the two VLCFAs, the O -acetylated one did not vary among all the lipid A species, while the other bearing the hopanoid residue was responsible for the observed heterogeneity in terms of length and hydroxylation pattern ( Figs 1b and 2 ). Although the occurrence of Bradyrhizobium species containing lipid A with two, three or even four VLCFAs has been already reported [19] , the presence of a hopanoid molecule covalently attached to lipid A had never been described in any LPS including those from non-photosynthetic Bradyrhizobium strains [19] , [20] , [21] , [22] . This represents a novel lipid A skeleton, which we name HoLA for Hopanoid-Lipid A. Analysis of hopanoid lipids present in Bradyrhizobium BTAi1 As most hopanoid-producing bacteria make a suite of hopanoids found within their inner and/or outer membranes [23] , [24] , [25] , [26] , we investigated the triterpenoid content of BTAi1 using GC-MS. Our data showed that it synthesized several hopanoids, including desmethyl and 2-methyl versions of diploptene, diplopterol and bacteriohopanetetrol ( Fig. 3 ). We were also able to detect BHP-550, which was most likely a degradation product of bacteriohopaneaminotriol. BTAi1 also produced tetrahymanol, a triterpenoid with a gammacerane skeleton. This indicated that BTAi1 possessed both ‘free’ and lipid A-bound hopanoids. 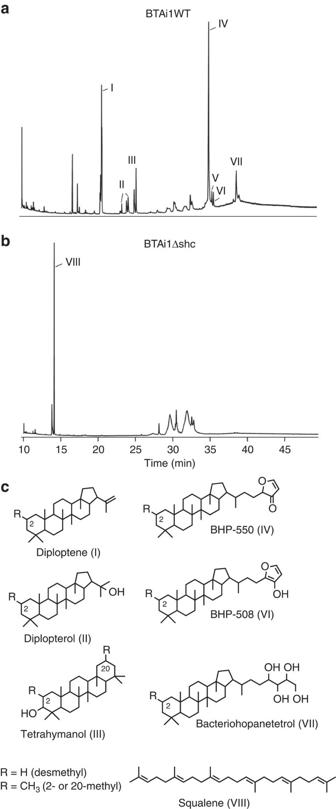Figure 3: GC-MS total ion chromatograms of acetylated total lipid extracts from BTAi1 strains. (a)Bradyrhizobiumstrain BTAi1 and (b)Bradyrhizobiumstrain BTAi1Δshc. Main hopanoid peaks are numbered and the 2-methyl counterparts elute 0.2–0.5 min earlier: I, diploptene (desmethyl and 2-methyl); II, diplopterol (desmethyl and 2-methyl); III, tetrahymanol (demethyl, 2-methyl and 20-methyl); IV, BHP-550; V, unidentified BHP; VI, BHP-508; VII, bacteriohopanetetrol (desmethyl and 2-methyl); VIII, squalene. Compounds were identified by comparison of retention times and mass spectra to those ofR. palustrisTIE-1 (ref.51). Lipid analysis for each strain was performed in triplicates. (c) Chemical structures of the isolated hopanoids. Figure 3: GC-MS total ion chromatograms of acetylated total lipid extracts from BTAi1 strains. ( a ) Bradyrhizobium strain BTAi1 and ( b ) Bradyrhizobium strain BTAi1Δ shc . Main hopanoid peaks are numbered and the 2-methyl counterparts elute 0.2–0.5 min earlier: I, diploptene (desmethyl and 2-methyl); II, diplopterol (desmethyl and 2-methyl); III, tetrahymanol (demethyl, 2-methyl and 20-methyl); IV, BHP-550; V, unidentified BHP; VI, BHP-508; VII, bacteriohopanetetrol (desmethyl and 2-methyl); VIII, squalene. Compounds were identified by comparison of retention times and mass spectra to those of R. palustris TIE-1 (ref. 51 ). Lipid analysis for each strain was performed in triplicates. ( c ) Chemical structures of the isolated hopanoids. Full size image Construction of a hopanoid-deficient mutant To investigate the biological significance of free as well as lipid A-bound hopanoids, we constructed a hopanoid minus mutant. A key step in the biosynthesis of hopanoids is the cyclization of the linear squalene into the pentacyclic triterpenoid hopene catalysed by squalene hopene cyclase (Shc) [27] . Genome sequence analysis of photosynthetic Bradyrhizobium strains revealed the presence of only one shc gene, which, in contrast to the non-photosynthetic strains, was not surrounded by other genes involved in hopanoid biosynthesis ( Supplementary Fig. 8a ). The hopanoid-deficient mutant (BTAi1Δ shc ) was constructed by deleting shc , and GC/MS analysis of the total lipid extract (TLE) confirmed that this mutant did not produce any type of hopanoid, including that linked to lipid A ( Fig. 3 ). In parallel, we isolated and purified LPS from Bradyrhizobium BTAi1Δ shc to check whether the mutation had any effect on lipid A structure. Our chemical, NMR and MS analyses showed that BTAi1Δ shc LPS was identical to BTAi1WT LPS, with the exception of the absence of the hopanoid substitution in the mutant ( Supplementary Fig. 9 ). This finding suggested that lipid A biosynthesis preceded its attachment to a hopanoid moiety. The enzyme(s) that catalyse(s) the covalent attachment of hopanoids to lipid A remain(s) to be discovered. Role of hopanoids in bacterial physiology As the absence of hopanoids in the membranes could modify their stability and therefore have a profound impact on BTAi1 physiology, we analysed the effect of the shc mutation on the growth of BTAi1 in both rich and minimal media. As shown in Fig. 4a,b , the growth rate of the mutant was markedly lower than that of the WT strain in both media. When we lowered the growth temperature to 30 or 25 °C to increase membrane stability, we still observed that the mutant grew less well than the WT; however, the difference in growth rates was less pronounced ( Supplementary Fig. 10 ). Notably, deletion of the shc gene in other bacteria, such as Rhodopseudomonas palustris TIE-1, a phylogenetically related species to photosynthetic bradyrhizobia, does not alter its growth rate at 30 °C under normal culture conditions [28] . 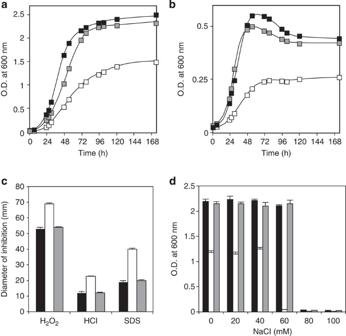Figure 4: Physiology of the hopanoid biosynthesis mutant (BTAi1Δshc). (a,b) Representative growth curves of BTAi1 (black square), BTAi1Δshc(white square) and complemented BTAi1Δshc+shc(grey square) strains cultivated in rich (a) or minimal medium (b). (c) Hydrogen peroxide (H2O2), hydrogen chloride (HCl) and sodium dodecyl sulfate (SDS) resistance of BTAi1 (black bar), BTAi1Δshc(white bar) and complemented BTAi1Δshc+shc(grey bar) strains, as determined by disk diffusion assays using 5 μl of 5.5 M H2O2, 2 N HCl or 10% of SDS according to a previously published protocol63. Error bars represent s.e. (n=9). (d) NaCl resistance of BTAi1 (black bar), BTAi1Δshc(white bar) and complemented BTAi1Δshc+shc(grey bar) strains. Error bars represent s.e. (n=3). Figure 4: Physiology of the hopanoid biosynthesis mutant (BTAi1Δ shc ). ( a , b ) Representative growth curves of BTAi1 (black square), BTAi1Δ shc (white square) and complemented BTAi1Δ shc+shc (grey square) strains cultivated in rich ( a ) or minimal medium ( b ). ( c ) Hydrogen peroxide (H 2 O 2 ), hydrogen chloride (HCl) and sodium dodecyl sulfate (SDS) resistance of BTAi1 (black bar), BTAi1Δ shc (white bar) and complemented BTAi1Δ shc+shc (grey bar) strains, as determined by disk diffusion assays using 5 μl of 5.5 M H 2 O 2 , 2 N HCl or 10% of SDS according to a previously published protocol [63] . Error bars represent s.e. ( n =9). ( d ) NaCl resistance of BTAi1 (black bar), BTAi1Δ shc (white bar) and complemented BTAi1Δ shc+shc (grey bar) strains. Error bars represent s.e. ( n =3). Full size image Hopanoids are thought to act as membrane condensers, thus increasing bacterial resistance to various abiotic stresses [6] , [29] , [30] , [31] . This prompted us to evaluate the ability of BTAi1Δ shc mutant to cope with various stressors. We tested oxidative, acid and detergent stresses using disk diffusion assays. Saline/osmotic stress was evaluated by comparing bacterial growth rates in the presence of increasing concentrations of NaCl. The data obtained ( Fig. 4c,d ) showed that the BTAi1Δ shc mutant was more sensitive than the WT strain to all stressors tested. Reintroduction of the shc gene under a constitutive promoter (P nptII ) into the Δ shc mutant restored growth and higher stress resistance under all conditions ( Fig. 4 ), excluding the possibility of polar effects or secondary mutation. These data indicated that hopanoids play an important role in the physiology of BTAi1. Role of hopanoids in symbiosis To determine whether hopanoids facilitate symbiosis, we infected the legume Aeschynomene evenia with both WT and Δ shc mutant BTAi1 strains and followed the kinetics of nodule formation. The complemented mutant was not tested during this experiment because the pMG103 plasmid used to reintroduce the shc gene was not stable in the BTAi1 strain in the absence of selective pressure and the spectinomycin antibiotic could not be used during plant culture. First observations were made after the symbiotic relationship had been well established with the formation of functional nodules [32] . At 6 days post inoculation (d.p.i. ), no significant differences were observed between plants inoculated with WT and mutant strains, the number of nodules per plants and the nitrogenase activity measured by the acetylene reduction assay (ARA) were comparable ( Fig. 5a,b ). This indicated that the Δ shc mutation had no effect on the ability of the bacteria to establish a symbiotic relationship. However, at 8 d.p.i., we observed that the plants inoculated with the Δ shc mutant fixed nitrogen slightly less efficiently than those inoculated with the WT strain, although the number of nodules elicited by the mutant was significantly higher ( Fig. 5a,b ). Cytological analysis of nodules (8 d.p.i.) using transmission electronic microscopy (TEM) revealed signs of nodule degeneracy. Although the endosymbiotic BTAi1Δ shc strain displayed, as did the WT, a typical spherical shape, indicating that the process of differentiation into bacteroids properly occurred, their size was smaller and the peribacteroid space was larger ( Fig. 5c–f ). Furthermore, some BTAi1Δ shc bacteroids displayed a profoundly perturbed envelope with a clear separation between the inner and outer membranes ( Fig. 5f ). Some bacteroids were far more drastically affected, with broken cell walls and an electron-dense cytoplasm suggesting that they were dead ( Fig. 5g ). At latter times (12 and 19 d.p.i. ), ARA activity of the plants inoculated with the mutant was only half that of plants inoculated with the WT strain, whereas twice more nodules per plant were formed with the mutant ( Fig. 5a,b ). This increase in the nodule number, similar to what had been observed upon infection with a nitrogenase minus mutant [33] , could be attributed to a phenomenon termed autoregulation of nodulation that ensures a balance between nodule formation and energy requirements in legumes [34] . At these times, we observed typical nitrogen starvation symptoms in the entire plant, for example, foliage chlorosis and reduced plant growth ( Fig. 5h ). These observations indicated that at early stages of the symbiotic interaction, the mutant was able to engage normally in an efficient association but that its nodules rapidly lost their ability to fix nitrogen. In agreement with this, at 19 d.p.i., the majority of the nodules elicited by the mutant were yellowish instead of green as observed for the WT nodules ( Fig. 5i,j ), hollow from inside ( Fig. 5k ), and did not display the red colour typical of leghaemoglobin as observed for the WT nodules ( Fig. 5l ). TEM observations showed no change in the ultrastructure of the WT nodules ( Fig. 5m ) in contrast to the mutant nodules for which the symbiotic tissues were digested ( Fig. 5n,o ). Such symptoms (leghaemoglobin degradation and symbiotic tissue digestion) characterize senescent nodules that occur naturally for WT nodules older than 50 days. 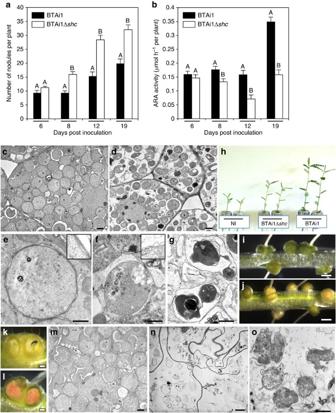Figure 5: The BTAi1Δshcmutant is severely impaired in symbiosis withA. evenia. (a) Nodulation kinetics ofBradyrhizobiumBTAi1 and BTAi1Δshcstrains onA. eveniaplants. (b) The occurrence of acetylene-reducing activity (ARA) inA. eveniaplants inoculated withBradyrhizobiumBTAi1 and BTAi1Δshcmutant. Error bars ina,brepresent s.e. (n=5). Different letters above the error bars indicate significant differences atP<0.05 (Tukey’s HSD test). (c–g) Transmission electron micrographs of nodules elicited by the WT strain (c,e) and the BTAi1Δshcmutant (d,f,g) at 8 d.p.i. Insets ine,fshow a detail of the cell wall ultrastructure of bacteroids. Scale bars are 1 μm (c,d), and 0.5 μm (e–g). (h) Comparison of the growth of the plants (aerial part) non-inoculated (NI) or inoculated with BTAi1 or BTAi1Δshcstrains (at 19d.p.i.). (i–l) Aspect of the nodules elicited by the WT strain BTAi1 (i,l) and the BTAi1Δshcmutant (j,k) at 19 d.p.i. Scale bars are 1 mm (i,j) and 100 μm (k,l). (m–o) Transmission electron micrographs of nodules elicited by the WT strain (m) and the BTAi1Δshcmutant (n,o) at 19 d.p.i. Scale bars are 1 μm (m,n) and 0.5 μm (o). Figure 5: The BTAi1Δ shc mutant is severely impaired in symbiosis with A. evenia . ( a ) Nodulation kinetics of Bradyrhizobium BTAi1 and BTAi1Δ shc strains on A. evenia plants. ( b ) The occurrence of acetylene-reducing activity (ARA) in A. evenia plants inoculated with Bradyrhizobium BTAi1 and BTAi1Δ shc mutant. Error bars in a , b represent s.e. ( n =5). Different letters above the error bars indicate significant differences at P <0.05 (Tukey’s HSD test). ( c – g ) Transmission electron micrographs of nodules elicited by the WT strain ( c , e ) and the BTAi1Δ shc mutant ( d , f , g ) at 8 d.p.i. Insets in e , f show a detail of the cell wall ultrastructure of bacteroids. Scale bars are 1 μm ( c , d ), and 0.5 μm ( e – g ). ( h ) Comparison of the growth of the plants (aerial part) non-inoculated (NI) or inoculated with BTAi1 or BTAi1Δ shc strains (at 19d.p.i.). ( i – l ) Aspect of the nodules elicited by the WT strain BTAi1 ( i , l ) and the BTAi1Δ shc mutant ( j , k ) at 19 d.p.i. Scale bars are 1 mm ( i , j ) and 100 μm ( k , l ). ( m – o ) Transmission electron micrographs of nodules elicited by the WT strain ( m ) and the BTAi1Δ shc mutant ( n , o ) at 19 d.p.i. Scale bars are 1 μm ( m , n ) and 0.5 μm ( o ). Full size image Together, these data showed that hopanoids play a critical role in chronic infection of the plant partner by BTAi1. Role of HoLA and free hopanoids in outer membrane stability To test the hypothesis that phenotypic defects observed both in planta and ex planta for the BTAi1Δ shc mutant resulted from the loss of integrity of the external membrane because of the lack of hopanoids, we analysed the ultrastructure of the WT strain and the BTAi1Δ shc mutant cultivated in free-living state using TEM. As shown in Fig. 6 , the WT cells were rod-shaped, with perfectly defined membranes, whereas the mutant cells displayed morphological distortion and an irregular outer boundary. These observations are consistent with outer membrane deformities previously reported for the Δ shc mutant of R. palustris TIE-1 (ref. 6 ). 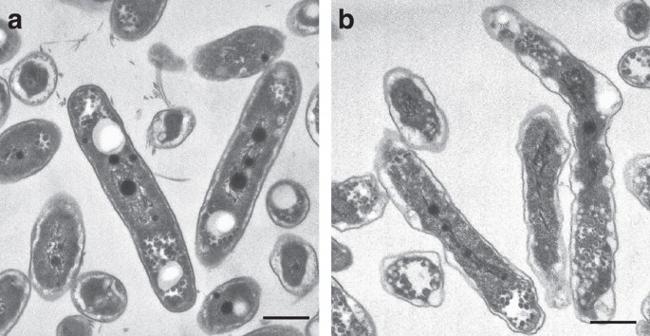Figure 6: The BTAi1Δshccells display membrane defects. (a,b) Transmission electron microscopy of BTAi1 (a) and BTAi1Δshc(b) cells grown on YM medium and harvested 120 h after inoculation. Scale bar, 0.5 μm. Figure 6: The BTAi1Δ shc cells display membrane defects. ( a , b ) Transmission electron microscopy of BTAi1 ( a ) and BTAi1Δ shc ( b ) cells grown on YM medium and harvested 120 h after inoculation. Scale bar, 0.5 μm. Full size image Furthermore, we investigated the microstructure of membranes from BTAi1 and the Δ shc mutant using ESR. We adopted a novel protocol for asymmetric liposome preparation based on the assembly of two independently prepared lipid monolayers (see Methods, Fig. 7a and Supplementary Note 5 ) [35] . In all cases, a unique distribution of liposome, whose dimension was centred at ~100 nm, was detected ( Supplementary Fig. 11 ). A phosphocholine spin-label on the 5 position of the acyl chain, 1-palmitoyl-2-[ 5 -(4,4 dimethyloxazolidine- N -oxyl)]stearoyl- sn -glycero-3-phosphocholine (5-PCSL), was included alternatively in the outer or in the inner lipid leaflet constituting the bilayer, thus allowing a direct detection of the lipid ordering and dynamics. 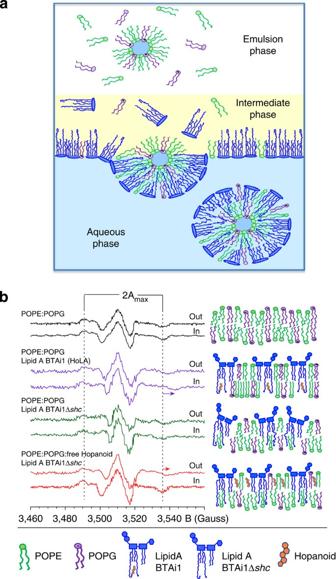Figure 7: Physicochemical characterization ofBradyrhizobiumBTAi1-reconstituted model membrane. (a) Schematic representation of asymmetric liposome formulation procedure. (b) ESR spectra of 5-PCSL in the outer (out) or inner (in) leaflet of the asymmetric liposomes whose components of the outer leaflet are specified in the figure. The inner leaflet is composed of a POPE/POPG mixture. A quantitative estimation of leaflet order and rigidity is obtained by determining the outer hyperfine coupling constant, 2Amax, as indicated in the figure. Increased 2Amax, as highlighted by the arrows, indicate higher order and/or rigidity. Sketches give a visual qualitative representation of the membranes. Figure 7: Physicochemical characterization of Bradyrhizobium BTAi1-reconstituted model membrane. ( a ) Schematic representation of asymmetric liposome formulation procedure. ( b ) ESR spectra of 5-PCSL in the outer (out) or inner (in) leaflet of the asymmetric liposomes whose components of the outer leaflet are specified in the figure. The inner leaflet is composed of a POPE/POPG mixture. A quantitative estimation of leaflet order and rigidity is obtained by determining the outer hyperfine coupling constant, 2 A max , as indicated in the figure. Increased 2 A max , as highlighted by the arrows, indicate higher order and/or rigidity. Sketches give a visual qualitative representation of the membranes. Full size image The ESR spectra showed evident perturbation in asymmetric bilayers including HoLA in the outer leaflet formulation ( Fig. 7b , Supplementary Table 4 ), indicating that HoLA insertion causes lower fluidity of the whole membrane, evocative of mechanical strengthening. In this respect, hopanoids serve the same function as sterols (for example, cholesterol) in eukaryotes [5] , [36] , although they appear to cause a weaker condensing and ordering effect [37] . Unexpectedly, the inner leaflet was even more affected by HoLA presence than the outer leaflet, in which lipid A had been positioned. This indicated that the long acyl chains of HoLA span both layers of the lipid membrane, so that the terminal hopanoid appendages were positioned in the inner leaflet ( Fig. 7b ). The result of this arrangement was twofold: (i) both leaflets were much more ordered and (ii) the leaflets were tightly linked, the long acyl chains acting as a ‘tightrope’ between the two membrane surfaces. We also studied asymmetric lipid bilayers including lipid A from the BTAi1Δ shc mutant in the outer leaflet formulation. In this case, the ESR spectra showed that the outer leaflet was less fluid than the inner one. Furthermore, the whole bilayer was less ordered than the one containing HoLA. This result indicated that linking the hopanoid moiety to the terminus of one acyl chain drove its insertion into the chains of the opposite leaflet. Finally, we considered a membrane whose outer leaflet contained the lipid A from the BTAI1Δ shc mutant and the hopanoid extract from Bradyrhizobium free of HoLA. The ESR spectra showed that only the outer leaflet was affected by the hopanoid-ordering effect, while the inner one remains almost unperturbed; this suggests that, in the absence of the covalent link to the long acyl chain, the hopanoid moiety tends to reside among the lipid A chains of the outer layer. These findings were supported by ESR results obtained using another spin-labelled lipid, 14-PCSL, bearing the radical reporter group on the 14 position of the acyl chain, thus monitoring the inner part of the bilayer hydrophobic core (see Supplementary Note 5 and Supplementary Fig. 12 ). It was found that HoLA was able to increase the acyl chain order in the whole membrane profile, including the central section. In conclusion, our results suggest that the molecular structure of HoLA is well suited to induce ordering of the asymmetric outer membrane, resulting in enhanced mechanical strength and stabilization. Hopanoids were described as abundant constituents of the membranes of Bradyrhizobium strains more than two decades ago. For instance, in B. diazoefficiens USDA110, they account for more than 40% of the total lipid fraction [3] . Despite the ecological and agricultural interest of these bacterial strains, we know relatively little about the structural and functional role of hopanoids. Besides the expected presence of ‘free’ hopanoids in the cell envelope of photosynthetic bradyrhizobia, here we discovered a novel LPS chemical architecture characterized by the covalent attachment of a hopanoid to the lipid A. Such LPS chemical architecture (HoLA) has not been described previously. Although we cannot ascertain the specific roles of HoLA compared with free hopanoids, our physical–chemical analyses, conducted on reconstituted asymmetric bilayers, clearly indicated that the HoLA molecules, spanning the whole outer membrane with the hopanoid located in the inner leaflet, permits a higher ordering and strengthening of both the inner and outer leaflets of the outer membrane, possibly imparting a functional advantage to the bacterium under some conditions. In detail, Bradyrhizobium BTAi1 synthesized a mixture of lipid A species differing by the number, length and nature of the acyl substitutions, linked or not to hopanoids. The availability of different types of lipid A could be an efficient strategy for BTAi1 to dynamically modulate the fluidity and rigidity of its outer membrane in response to environmental changes. Several interesting phenotypes arose from the absence of hopanoids in photosynthetic bradyrhizobia. These included growth defects in the presence of different stressors, and an inability to maintain a chronic intracellular infection in a symbiotic context. In the intracellular milieu of the legume cell, the rhizobium has to cope with various stresses such as peribacteroid space acidification [38] and oxidative stress because of the production of reactive oxygen and nitrogen species (H 2 O 2 , O 2 − and NO) by the host cell [39] . In addition, recent data suggested that Aeschynomene use antimicrobial peptides similar to NCR peptides described in Medicago to control bacteroid differentiation [40] . It is known that shc mutants of some bacterial species are more sensitive to these compounds [41] , [42] . It could be therefore possible that the symbiotic deficiency of the shc mutant resulted from its inability to survive in such a harsh intracellular environment. Identifying the enzyme(s) that catalyse(s) the attachment of hopanoid to lipid A will enable the precise role of HoLA to be determined as well as allow us to assess the phylogenetic distribution of HoLA among Gram-negative bacteria, assuming that this enzyme is well conserved. In R. palustris , a bacterium closely related to Bradyrhizobium , all the genes involved in hopanoid biosynthesis are located close together in a DNA region called the hopanoid biosynthetic gene cluster [28] . This cluster is well conserved in all Bradyrhizobium strains; however, in photosynthetic bradyrhizobia, the shc gene was found elsewhere in the genome. Besides the fact that the gene organization surrounding shc is different, phylogenetic analysis showed that shc genes from photosynthetic and non-photosynthetic Bradyrhizobium form two distant clusters ( Supplementary Fig. 8b ). A high level of identity was observed between the Shc proteins belonging to the same clade (> at 85%), whereas this identity dropped to only 35% between Shc proteins belonging to different clades. Altogether, these data suggested that the two classes of Shc could have different biochemical properties and functional roles, which could be related to the ability to synthesize HoLA. Experiments are in progress to exchange the shc genes between photosynthetic and non-photosynthetic bradyrhizobia to clarify the specific roles of these two Shc types by analysing the impact of this allelic exchange on LPS structure and hopanoid content. In summary, the discovery that HoLA and hopanoids contribute to the outer membrane structure of photosynthetic bradyrhizobia could have important biotechnology applications. For instance, manipulation of hopanoid biosynthesis could be used either to strengthen this barrier, thus increasing the ability of bacteria to survive stress conditions, or to relax this barrier, thus promoting the exchange of diffusible molecules between the bacteria and the external environment. Future studies will shed light on the specific mechanisms, whereby hopanoids and HoLA enhance cell membrane properties in the context of plant–microbe symbioses. Bacterial strains and growth conditions Bradyrhizobium strain BTAi1 and derivatives (BTAi1Δ shc and BTAi1Δs hc+shc ) were grown in rich YM medium [43] or BNM (buffered nodulation medium) minimal medium [44] at 37 °C. When required, the media were supplemented with kanamycin (50 μg ml −1 ) for BTAi1Δ shc and a mixture of kanamycin (50 μg ml −1 ) and spectinomycin (50 μg ml −1 ) for BTAi1Δs hc+shc . Recovery of LPS from Bradyrhizobium BTAi1 and BTAi1Δ shc In order to recover the LPS material, bacterial cells were extracted applying the phenol/water method [45] and, after extensive dialyses, the extracted phases were subjected to a step of enzymatic digestions with DNAse, RNAse and protease in order to remove nucleic acid and protein contaminants and recovered using ultracentrifugation (100,000 g , 4 °C, 24 h). Both water and phenol fractions were analysed through SDS–polyacrylamide gel electrophoresis (SDS–PAGE) 13.5%; the LPS fraction was exclusively found in the water phase as suggested by the presence of the typical ladder in its migration pattern in the gel ( Supplementary Fig. 13 ). The LPS fraction was further purified using size filtration chromatography (SephacrylS-400 HR in 50 mM (NH 4 ) 2 CO 3 from GE Healthcare; yield 3% of dried material). Compositional analysis Sugar content was determined with the GC-MS analysis of acetylated O -methyl derivatives. The dried LPS sample was left over a drying agent, under continuous vacuum, for a couple of hours. Then 1 ml of methanolic HCl was added and incubated at 85 °C for 16 h, the sample was dried in a stream of air, subsequently acetylated extract with pyridine (25 μl) and Ac 2 O (25 μl), 80 °C, 30 min and analysed using gas-liquid cromatography (GLC)-MS [46] . Linkage analysis was carried out by methylation of the complete core region as described. The sample was hydrolysed with 4 M trifluoroacetic acid (100 °C, 4 h), carbonyl-reduced with NaBD 4 , carboxy-methylated, carboxyl-reduced, acetylated and analysed using GLC-MS [47] . Total fatty acid content was obtained by acid hydrolysis. LPS was first treated with 4 M HCl (4 h, 100 °C) and then with 5 M NaOH (30 min, 100 °C). Fatty acids were then extracted in CHCl 3 , methylated with diazomethane and analysed using GLC-MS. The ester-bound fatty acids were selectively released by base-catalysed hydrolysis with 0.5 M NaOH/MeOH (1:1 v/v, 85 °C, 2 h), and then the product was acidified, extracted in CHCl 3 , methylated with diazomethane and analysed using GLC-MS [48] . Recovery of lipid A from Bradyrhizobium BTAi1 and BTAi1Δ shc In order to obtain lipid A, LPS was dissolved in acetate buffer (pH 4.4) and the hydrolysis was run for 5 h at 100 °C. It was purified according to the procedure provided in ref. 49 . In brief, adequate amounts of chloroform and methanol were added to the hydrolysate to obtain chloroform/methanol/hydrolysate 2:2:1.8 (v/v/v), and the mixture was vigorously shaken, and then centrifuged. The chloroform phase, containing the lipid A, was collected and washed twice with the water phase from a freshly prepared two-phase Bligh/Dyer mixture (chloroform/methanol/water, 2:2:1.8 (v/v/v)) [50] . The organic phases were collected and dried. Recovery of hopanoid extracts In order to recover hopanoid lipids, bacterial cells from Bradyrhizobium were extracted as follows [3] , [50] . WT and Δ shc cultures were grown in triplicates in 2-l flasks with 200 ml YM medium at 37 °C in dark for ca. 72 h. Cultures were harvested using centrifugation at 5,000 g for 15 min at 4 °C and the cell pellets frozen at −80 °C until ready for use. Lipid extraction was performed by resuspending cells in 6 ml of water, 2 ml of which were transferred into Teflon centrifuge tubes (VWR, Bridgeport, NJ). This was followed by addition of 5 ml of methanol (MeOH) and 2.5 ml of dichloromethane (DCM) and sonication for 15 min at room temperature. Samples were centrifuged at 7,000 g for 10 min at 22 °C and the supernatants were transferred to new tubes. The cell pellets were resuspended again in 9.5 ml of 10:5:4 MeOH:DCM:H 2 O, sonicated and centrifuged and the supernatants were combined with the first extraction. The samples were separated into two phases by adding ~13 ml of DCM and centrifuging at 6,000 g for 10 min at 22 °C. The lower organic phase was transferred to a new glass vial and evaporated in a chemical hood overnight (TLE). The TLE was resuspended in DCM at a concentration of 1 mg ml −1 . Hundred microlitres of this extract was evaporated under 60 °C and then derivatized to acetate esters by incubation in 100 μl of 1:1 acetic anhydride:pyridine for 30 min at 60 °C. The acetylated TLEs were analysed using high-temperature GC-MS [51] . Compounds were identified by comparison of retention times and mass spectra with those of R. palustris TIE-1 (ref. 6 ). NMR spectroscopy NMR spectra of the lipid A fraction were recorded in CDCl 3 /MeOD 1:1 at 25 °C, on Bruker 600 DRX equipped with a cryo probe. ROESY (rotating-frame Overhauser effect spectroscopy) and NOESY (nuclear Overhauser effect spectroscopy) experiments were recorded using data sets (t1 × t2) of 4,096 × 256 points with mixing times at 100–200 ms. Double quantum-filtered phase-sensitive COSY (double quantum-filtered Correlation SpectroscopY) experiments were performed using data sets of 4,096 × 512 points. TOCSY (Total Correlation Spectroscopy) experiments were performed with spinlock times of 100 ms, using data sets (t1 × t2) of 4,096 × 256 points. In all homonuclear experiments, the data matrix was zero-filled in both dimensions to give a matrix of 4 K × 2 K points and was resolution-enhanced in both dimensions by a cosine-bell function before Fourier transformation. Coupling constants were determined by two-dimensional (2D) phase-sensitive DQF-COSY [52] , [53] . HSQC (Heteronuclear Single Quantum Correlation), J -coupled HSQC, HSQC-TOCSY and HMBC (Heteronuclear Multiple-Bond Correlation) experiments were measured in the 1 H-detected mode via single quantum coherence with proton decoupling in the 13 C domain, using data sets of 2,048 × 256 points. Experiments were carried out in the phase-sensitive mode [54] . A 60-ms delay was used for the evolution of long-range connectivities in the HMBC experiment. In all heteronuclear experiments, the data matrix was extended to 2,048 × 1,024 points using forward linear prediction extrapolation. MALDI TOF MS This study used a 4,800 Proteomic Analyzer (ABSciex), MALDI TOF/TOF (time of flight, TOF) instrument equipped with a Nd:YAG laser at a wavelength of 355 nm with <500-ps pulse and 200-Hz firing rate. External calibration was performed using an ABSciex calibration mixture. Mass accuracy was about 55 p.p.m. All measurements were performed in positive polarity. Approximately, 1,500 laser shots were accumulated for each spectrum in the MS experiments; 5,000–7,000 shots were summed for the MS/MS data acquisitions [55] , [56] . The tandem mass spectra reported in this study were acquired without a collision gas. Samples were dissolved in CHCl 3 /CH 3 OH (50:50, v/v) at a concentration of 1 mg ml −1 . Matrix solution was prepared by dissolving trihydroxyacetophenone in CH 3 OH/0.1% trifluoroacetic acid/CH 3 CN (7:2:1, by volume) at a concentration of 75 mg ml −1 . One microlitre of the sample/matrix solution (1:1, v/v) was deposited on the well plate and allowed to dry at room temperature [57] . ESR and DLS studies of lipid A-containing membranes Asymmetric liposomes were prepared assembling two independently prepared lipid monolayers. The inner one consisted of a 70/30 mol/mol mixture of 1-palmitoyl-2-oleoyl- sn -glycero-3-phosphoethanolamine (POPE) and 1-palmitoyl-2-oleoyl- sn -glycero-3-phospho-(1′- rac -glycerol) (POPG). In the outer one, 75% by mass of the POPE–POPG lipid mixture was substituted with HoLA (or its BTAi1Δ shc mutant). In some formulations, free hopanoid was also included. POPE and POPG were obtained from Avanti Polar Lipids (Birmingham, AL, USA) and used without further purification. The spin-labelled phosphatidylcholines (1-palmitoyl-2-[ n -(4,4 dimethyloxazolidine- N -oxyl)]stearoyl- sn -glycero-3-phosphocholine, n -PCSL, n =5, 14), used for ESR measurements, were also purchased from Avanti Polar Lipids and stored at −20 °C in ethanol solutions. The liposome preparation procedure is schematized in Fig. 7a . The inner leaflet resulted from a W/O emulsion (the ‘emulsion phase’ in the Fig. 7a ) which was prepared, in turn, from a lipid suspension. To prepare the lipid suspension, 80 μl of a 25-mg ml −1 POPE/POPG (70/30 mol/mol) stock solution in chloroform were placed in a 100-ml glass bottle. The chloroform was evaporated under nitrogen to obtain a dry, thin lipid film. After adding 4 ml of anhydrous dodecane (>99%) to reach a final lipid concentration of 0.5 mg ml −1 , the suspension was sonicated in a cleaning sonic bath for 45 min and left overnight at 25 °C to ensure that the lipid molecules were fully dispersed in oil before emulsifying the aqueous solution. The emulsion was prepared by adding 200 μl of an aqueous 10 mM phosphate buffer at pH=7.4, containing 1 mM Ca 2+ , to the lipid suspension and gently stirring the mixture with a magnetic stir bar for 1 h. Finally, the emulsion was sonicated using a tip probe for 20 min in an ice bath. Droplets’ dimension distribution was checked by DLS (see Supplementary Fig. 11 ) to be monomodal, centred at ~130 nm. DLS analysis was performed with a set-up composed by a Photocor compact goniometer, a SMD 6000 Laser Quantum 50 mW light source operating at 5,325 Å and a PMT-120-OP/B and a correlator (Flex02-01D, Correlator.com). The outer leaflet of the liposome was obtained from a lipid monolayer stratified at the interface between a phosphate buffer (the ‘aqueous phase’ in the figure) and a lipid organic mixture (the ‘intermediate phase’). To prepare this organic mixture the chosen lipid A, POPE and POPG at the proper ratio were dispersed at a concentration of 0.2 mg ml −1 in a toluene/silicone oil (99/1 mol/mol) solution. One millilitre of this lipid dispersion was slowly placed over 0.6 ml of Ca 2+ -containing phosphate buffer in a centrifuge tube, waiting 24 h to allow the neat stratification of the organic phase over the aqueous medium and the formation of a lipid monolayer at the interface. Once the interface had equilibrated, 100 μl of the W/O emulsion was gently poured over the organic phase. Then the sample was centrifuged at 3,500 g for 10 min to transfer the water droplets through the interface and into the lower aqueous phase, see Fig. 7a . After centrifugation, the aqueous phase containing the liposomes was collected using a 5-ml syringe with a long stainless steel needle. Formation and dimension of obtained liposomes were assessed using DLS ( Supplementary Fig. 11 ) and the mean hydrodynamic radius was found to be 180 and 190 nm with BTAi1Δshc and HoLA, respectively. For ESR measurements, each liposome sample to be investigated was prepared twice, and the 5-PCSL spin-label was alternatively added to the inner (3% wt/wt on the total lipid) or outer lipid leaflet (1% wt/wt on the total lipid) by mixing appropriate amounts of a spin-label solution in ethanol (1 mg ml −1 ) with either the POPE–POPG solution in chloroform or the lipid A dispersion in toluene/silicone oil. In a separate set of experiments, the 14-PCSL spin-label was added to the inner leaflet by using the same procedure used for the 5-PCSL spin-label. Four liposome formulations were considered (that is, eight samples were prepared): (1) symmetric POPE–POPG liposomes, used as a reference; (2) asymmetric liposomes with the external leaflet formed by a HoLA–POPE–POPG mixture and the inner leaflet formed by POPE–POPG; (3) asymmetric liposomes with the external leaflet formed by a BTAi1Δ shc lipid A–POPE–POPG and the inner leaflet formed by POPE–POPG; (4) asymmetric liposomes with the external leaflet formed by the BTAi1Δ shc lipid A, the inner leaflet formed by POPE–POPG and the hopanoid extract, at the same mole ratio of BTAi1, added to the toluene/silicone oil mixture. ESR spectra of 5-PCSL and 14-PCSL in the considered samples were recorded on a Elexys E-500 ESR spectrometer from Bruker (Rheinstetten, Germany) operating in the X band. Capillaries containing the samples were placed in a standard 4-mm quartz sample tube. The temperature of the sample was regulated at 30 °C and maintained constant during the measurement by blowing thermostated nitrogen gas through a quartz Dewar. Samples containing the 5-PCSL spin-label in the inner leaflet were also investigated in a temperature range spanning from 15 to 45 °C. The instrumental settings were as follows: sweep width, 120 G; resolution, 1,024 points; modulation frequency, 100 kHz; modulation amplitude, 1.0 G; time constant, 20.5 ms; sweep time, 42 s; incident power, 5.0 mW. Several scans, typically 16, were performed and averaged to improve the signal-to-noise ratio. Construction of the BTAi1Δ shc mutant and complementation To create the BTAi1Δ shc mutant, the complete shc gene was deleted and replaced by the kanamycin-resistance (KnR) gene by double crossover recombination as described below. The KnR gene was under the control of its own promoter and no termination sequence was introduced downstream this gene. A 2,331-bp shc gene fragment including 99-bp upstream and 177-bp downstream regions was amplified using the primers SHCFW (5′-CGCTACGGCCAGTTGATTGGATTT-3′) and SHCRV (5′-TGCATCCGAAGCTCAGGACAATGA-3′) and cloned into pGEM-T easy vector (Promega Corp., Madison, WI, USA). The resulting plasmid was named pGEM-T:: shc . The NotI fragment sized ca. 2.4 kb digested from pGEM-T:: shc was ligated with NotI-digested pJQ200SK [58] that is not replicable in Rhizobium species, and which contains a counter selectable sac B marker, resulting in pJQ:: shc . This pJQ:: shc was introduced into DH5α (pKD78), which has λ Red recombinase gene controlled by araBAD promoter, by electroporation. The kanamycin-resistance gene was amplified from pKD4 (ref. 59 ) using the primers PS1 (5′-GTGTAGGCTGGAGCTGCTTC-3′) and PS2 (5′-CATATGAATATCCTCCTTAG-3′). Using the PCR product as a template, the kanamycin-resistance gene was re-amplified with two 60-bp primers PSHC1 and PSHC2, which have 40-bp linkers homologous to both bordering regions of the shc gene at 5′ ends of PS1 and PS2. The sequences of PSHC1 and PSHC2 are 5′-GCCCTGCAATCGACGGTGCGCGCGGCGGCGGATTGGCTGAGTGTAGGCTGGAGCTGCTTC-3′ and 5′-GTACATGCCGTAGCGGAGCATGAAGGCGCGGGACAATTCCCATATGAATATCCTCCTTAG-3′, respectively. The consequent PCR product was introduced into DH5α (pKD78/pJQ:: shc ) and the λ Red recombinase was induced [60] . The resulting plasmid named pShc::Km was transferred into BTAi1 by triparental mating [60] and the shc gene replacement in sucrose-resistant clones was confirmed using PCR. For complementation of the mutant, the complete shc gene was cloned downstream of the nptII promoter into the pMG103-npt2-GFP plasmid [61] harbouring a streptomycin/spectinomycin-resistance gene. For this, the streptomycin/spectinomycin-resistance gene was first liberated from pHRP315 (ref. 62 ) by BamHI digestion and cloned into the corresponding site of pMG103-npt2-GFP; the shc gene amplified using the primers SHC-BTAi1-F (5′-GGCGGAGATCTTCCCTATAGGGCGGGGTGAATTC-3′) and SHC-BTAi1-R (5′-CCGTCACTAGTCGCGCGACGGGATGGCTCGCAATG-3′) was then cloned into the BglII/SpeI sites located downstream of the nptII promoter. Plant cultivations and symbiotic analysis A. evenia seeds were surface-sterilized by immersion in sulphuric acid under shaking during 40 min. Seeds were abundantly washed with sterile distilled water and incubated overnight in sterile water. Seeds were then transferred for 1 day at 37 °C in darkness on 0.8% agar plate for germination. Plantlets were then transferred on the top of test tubes covered by aluminium paper for hydroponic culture in BNM. Plants were grown in closed mini green house in a 28 °C growth chamber with a 16-h light and 8-h dark regime and 70% humidity. Seven days after transfer, each seedling was inoculated with 1 ml of cell suspension resulting from a 5-day-old bacterial culture washed in BNM and adjusted to reach an optical density of one at 600 nm. For nodulation and nitrogen fixation kinetics at different times post inoculation (6, 8, 10, 12 and 19 days), five plants were taken to count the number of nodules on the roots and to analyse the nitrogenase activity by ARA. For this, each plant was placed into 125-ml glass vials sealed with rubber septa. Air (12.5 ml) was removed from each vial, to which 12.5 ml of acetylene was then injected. Gas samples (1 ml) were withdrawn after 3 h of incubation at 25 °C and the ethylene produced was measured using gas chromatography. Transmission electron microscopy Microscopic observations were performed on three to five nodules originating from different plants per condition. For this, the nodules were fixed in a 4% glutaraldehyde, 0.1 M cacodylate buffer (pH 7.2), postfixed in 1% osmium tetroxide, dehydrated using a series of acetone washes and embedded in TAAB 812 epon resin. Ultrathin sections (60 nm) were mounted on collodion carbon-coated copper grids, contrasted using uranyl acetate and lead citrate and examined at 80 kV with a TEM (Jeol 100CX II). How to cite this article: Silipo, A. et al. Covalently linked hopanoid-lipid A improves outer-membrane resistance of a Bradyrhizobium symbiont of legumes. Nat. Commun. 5:5106 doi: 10.1038/ncomms6106 (2014).